The synergetic effect of lithium polysulfide and lithium nitrate to prevent lithium dendrite growth Lithium metal has shown great promise as an anode material for high-energy storage systems, owing to its high theoretical specific capacity and low negative electrochemical potential. Unfortunately, uncontrolled dendritic and mossy lithium growth, as well as electrolyte decomposition inherent in lithium metal-based batteries, cause safety issues and low Coulombic efficiency. Here we demonstrate that the growth of lithium dendrites can be suppressed by exploiting the reaction between lithium and lithium polysulfide, which has long been considered as a critical flaw in lithium–sulfur batteries. We show that a stable and uniform solid electrolyte interphase layer is formed due to a synergetic effect of both lithium polysulfide and lithium nitrate as additives in ether-based electrolyte, preventing dendrite growth and minimizing electrolyte decomposition. Our findings allow for re-evaluation of the reactions regarding lithium polysulfide, lithium nitrate and lithium metal, and provide insights into solving the problems associated with lithium metal anodes. Lithium metal, having a high theoretical specific capacity of 3,860 mAh g −1 and the most negative electrochemical potential among anode materials, has been considered an ideal anode in lithium battery systems over the past four decades [1] , [2] , [3] , [4] , [5] , [6] . The recent emerging demand for extended-range electric vehicles has stimulated the development of high-energy storage systems [7] , [8] , [9] , [10] , especially the highly promising lithium–sulfur and lithium–air batteries, in which lithium metal anodes are employed. However, practical applications of rechargeable lithium metal-based batteries have been hindered by the formation of dendritic and mossy lithium and associated electrolyte decomposition, resulting in safety concerns and low Coulombic efficiency [11] , [12] . Uncontrolled growth of lithium dendrites originates from the repeated stripping/plating of a lithium layer during cycling [2] , [5] , [11] , [12] , [13] , associated with which is a large volume change that causes cracks in the solid-electrolyte interphase (SEI) that exposes fresh lithium metal to the electrolyte, resulting in continuous electrolyte decomposition and rapid loss of both working lithium and electrolyte. The SEI formation is spatially inhomogeneous because of this volume change and thus causes non-uniform lithium deposition across the electrode, further aggravating the growth of dendritic lithium. Therefore, the formation of a SEI layer with high uniformity and stability is essential to ensure high Coulombic efficiency, long cycle life and safety in lithium metal-based batteries. Among various approaches to overcoming the issues of lithium metal anode, it is recognized that electrolyte selection is one of the most dominant factors for stabilizing the lithium metal surface [14] , [15] , [16] , [17] , [18] , [19] , [20] , [21] , [22] , [23] , [24] , [25] , [26] , [27] . Although various polymeric and ceramic electrolytes have been demonstrated to suppress lithium dendrite growth [14] , [15] , [16] , [17] , [18] , [19] , [20] , their ionic conductivity, interfacial impedance, mechanical moduli or chemical stability when in contact with metallic lithium were not satisfying and still need further improvement for their implementation. In liquid electrolytes, many additives including organic and inorganic compounds have been used to improve the stability of the SEI layer [21] , [22] , [23] , [24] , [25] . However, the low solubility of many additives in the electrolyte and their rapid consumption during cycling undermines their effectiveness in suppressing dendrite growth. Thus, the SEI layers in previous studies were still not able to maintain their integrity during long-term cycling. Besides adding additives that are soluble in the electrolyte, Archer’s group demonstrated the use of hybrid electrolytes containing solid particles, such as ionic liquid–nanoparticle hybrid electrolytes, and liquid electrolytes reinforced with halogenated salt solid blends, to retard lithium dendrite growth and exhibit stable cycling in carbonate electrolyte [26] , [27] , [28] . Recently, Xu and coworkers [29] proposed a self-healing electrostatic shielding mechanism using alkaline ion additives in carbonate electrolyte that could in principle prevent dendrite formation without consuming the additives. However, the Coulombic efficiency of 76.6% suggests that continuous reaction of lithium with the electrolyte is not avoided. Previous research of screened different electrolyte compositions suggest that ether-based electrolytes, which are commonly used in high-energy lithium–sulfur and lithium–air battery systems, could be better choices for lithium metal-based batteries [30] . Compared with the carbonate electrolytes that are used in commercial lithium–ion batteries, the SEI formed in ether-based electrolyte comprises oligomers that have a certain extent of flexibility, which can better accommodate the volume change of the lithium anode [30] , [31] . Most recently, our group developed a nanoscale interfacial engineering approach for lithium anodes by coating a monolayer of interconnected hollow carbon spheres or ultrathin two-dimensional layers of boron nitride and graphene on the lithium metal surface [32] , [33] , which can suppress dendrite growth and facilitate the formation of a stable SEI. However, the Coulombic efficiency at high current density/capacity still needs further improvement. The exploration of appropriate electrolyte additives to stabilize the interface between lithium metal and electrolyte is a simpler approach that could be most easily adapted to practical applications. For lithium metal anode, an ideal electrolyte additive should react with lithium to a certain extent forming a strong and chemically stable SEI layer, but should not be too reactive to avoid consuming too much lithium. Long-chain lithium polysulfides (Li 2 S x , 4≤ x ≤8) are intermediate reaction species generated from the sulfur cathode during charge/discharge process of typical lithium–sulfur batteries [8] , [34] , [35] , [36] . These polysulfide ions are highly soluble in ether-based electrolytes and can diffuse to the anode side where they react with lithium to be reduced to short-chain lithium polysulfides (Li 2 S x , 1≤ x ≤3). This reaction can cause active mass loss of sulfur cathodes and has long been considered the main reason for rapid capacity decay of lithium–sulfur batteries. Herein, we demonstrate that the parasitic reaction between lithium polysulfide and lithium can instead be used to effectively suppress the growth of lithium dendrites. Both lithium polysulfide (Li 2 S 8 ) and lithium nitrate (LiNO 3 ) were used as additives to the ether-based electrolyte, which enables a synergetic effect leading to the formation of a stable and uniform SEI layer on lithium surface that can greatly minimize the electrolyte decomposition and prevent dendrites from shooting out. By simply manipulating the concentrations of Li 2 S 8 and LiNO 3 , we show that the formation of lithium dendrites can be prevented at a practical current density of 2 mA cm −2 up to a deposited areal capacity of 6 mAh cm −2 . We also demonstrate excellent cyclability: the Coulombic efficiency can be maintained at >99% for over 300 cycles at 2 mA cm −2 with a deposited capacity of 1 mAh cm −2 . Even for cyclic deposition of a high areal capacity of 3 mAh cm −2 , the average Coulombic efficiency can be as high as 98.5% over 200 cycles (and is higher at ∼ 99.0% between 70 and 200 cycles). In addition, using in-situ optical imaging, we were able to observe that the polysulfide additive smooths the lithium dendrites through an etching effect. This provides us valuable insight in understanding the structural evolution of the lithium anode. Morphology of lithium metal deposition We investigated the process of lithium metal plating/stripping using a two-electrode configuration composed of a lithium metal electrode and a stainless steel foil (substrate for lithium plating/stripping), assembled in 2,032-type coin cells. The electrolyte was 1.0 M LiTFSI (lithium bis(trifluoromethanesulfonyl)imide) in 1,3-dioxolane and 1,2-dimethoxyethane (volume ratio 1:1). A constant current is applied to the electrodes while the potential is recorded versus time. A fixed amount of lithium (calculated based on the capacity) was first deposited onto the stainless steel substrate, followed by subsequent lithium dissolution and re-deposition. 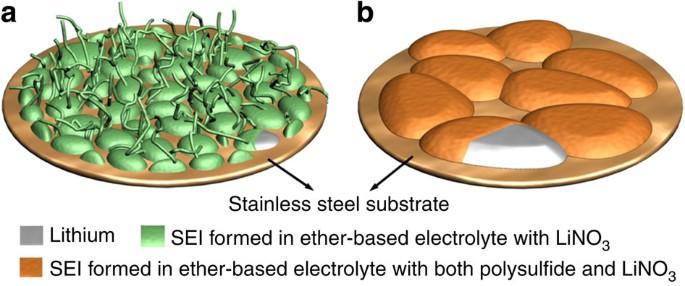Figure 1: Schematic of the morphologies of lithium deposited on the substrate in different electrolytes. Schematic illustration showing the morphology difference of lithium deposited on the stainless steel substrate in the two electrolytes (both contain lithium nitrate), but (a) without lithium polysulfide (b) containing lithium polysulfide. Figure 1 schematically illustrates the morphology difference of the lithium deposited on the stainless steel substrate in the electrolytes with and without lithium polysulfide (both electrolytes contain LiNO 3 ; the corresponding experimental results are shown in Fig. 2 ). As shown in Fig. 1a , the SEI layer formed is not mechanically strong enough to accommodate the volume expansion on lithium plating, creating cracks and pits with lower impedance. Therefore, lithium preferentially deposits at these defect sites, causing rapid growth of lithium filaments and dendrites. In contrast, when polysulfide (Li 2 S 8 ) is added to the electrolyte, fewer nucleation sites of lithium are generated in the initial stage of the deposition due to the reaction between Li 2 S 8 and lithium. This contributes to the subsequent growth of lithium with pancake-like morphology that has much smaller surface area ( Fig. 1b ), enabling the formation of a stable and uniform SEI on the lithium surface that can prevent the growth of dendritic lithium. Figure 1: Schematic of the morphologies of lithium deposited on the substrate in different electrolytes. Schematic illustration showing the morphology difference of lithium deposited on the stainless steel substrate in the two electrolytes (both contain lithium nitrate), but ( a ) without lithium polysulfide ( b ) containing lithium polysulfide. 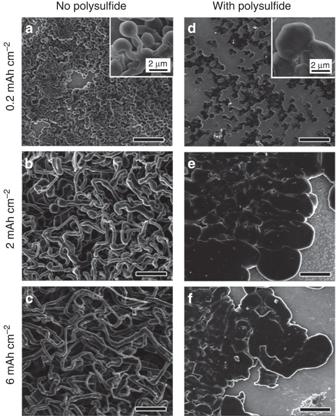Figure 2: Morphology characterization of lithium metal deposited onto stainless steel substrate. SEM images of lithium metal deposited onto bare stainless steel substrate (the edge region of the whole deposition area) in the electrolyte (a–c) with the addition of only LiNO3(1 wt%) and (d–f) with the addition of both Li2S8(0.18 M) and LiNO3(1 wt%) at a current density of 2 mA cm−2and deposition capacities of 0.2, 2 and 6 mAh cm−2, respectively. Scale bars, 20 μm. Full size image Figure 2: Morphology characterization of lithium metal deposited onto stainless steel substrate. SEM images of lithium metal deposited onto bare stainless steel substrate (the edge region of the whole deposition area) in the electrolyte ( a – c ) with the addition of only LiNO 3 (1 wt%) and ( d – f ) with the addition of both Li 2 S 8 (0.18 M) and LiNO 3 (1 wt%) at a current density of 2 mA cm −2 and deposition capacities of 0.2, 2 and 6 mAh cm −2 , respectively. Scale bars, 20 μm. Full size image Previous modelling of lithium deposition showed that for planar electrodes, lithium deposition preferentially occurs at the edges of the electrode due to the greater accessibility of electrolyte to the edge region than the centre part (higher concentration of lithium ion flux at the edge region) [37] . In our experiments, we found correspondingly that the deposited lithium at its edge area, where lithium can grow unimpeded by the constraint of the separator and opposing electrode, exhibited a much more dendritic morphology than the lithium deposited in the centre portion. Therefore, the influence of the different electrolytes on the morphology of the deposited lithium was much more pronounced at the edge areas and is emphasized in the results that follow. Figure 2 shows scanning electron microscopy (SEM) images of lithium metal deposited onto the bare stainless steel substrate (the edge region of the whole deposited area) for the electrolyte with addition of only LiNO 3 ( Fig. 2a–c ) and for the addition of both Li 2 S 8 and LiNO 3 ( Fig. 2d–f ), at a current density of 2 mA cm −2 and a deposition capacity of 0.2, 2 and 6 mAh cm −2 . It has been reported that for lithium–sulfur batteries, the Coulombic efficiency can be greatly improved by adding LiNO 3 to the electrolyte to minimize the shuttle effect of lithium polysulfides [31] , [38] . Here we found that the LiNO 3 additive alone also has an effect on lithium dendrite morphology. Much sharper, thinner and fibre-like lithium dendrites were formed when no LiNO 3 was present ( Supplementary Fig. 1 ) compared with the thicker, less sharper morphology of lithium filaments deposited in the electrolyte with LiNO 3 ( Fig. 2b ). However, LiNO 3 alone is not sufficient to prevent dendrite growth. For the electrolyte using only LiNO 3 as additive, it can be observed that filaments grow out from the granular lithium particles ( Fig. 2a ) when the deposition capacity is as low as 0.2 mAh cm −2 . As lithium continues to deposit, more lithium filaments with longer and sharper morphology are observed ( Fig. 2c ). These structures not only threaten the safety of batteries by penetrating through the separator, but also contribute to a higher possibility of dead lithium on stripping. In comparison, when both Li 2 S 8 and LiNO 3 were added to the electrolyte, at low deposited capacity (0.2 mAh cm −2 ), a lower density of nucleated lithium particles was formed ( Fig. 2d ), which can be attributed to a competition between etching and deposition of lithium. Subsequent lithium plating leads to the formation of lithium having a pancake-like morphology with much lower surface area ( Fig. 2e ) than seen with LiNO 3 alone. Even at a high deposition capacity of 6 mAh cm −2 , no long filaments or dendrites were observed ( Fig. 2f ). The same morphology trends for the two electrolytes were found for the lithium metal deposited onto the centre regions of the stainless steel substrates ( Supplementary Fig. 2 ). Moreover, the top surface of the plated lithium (the edge region) after 100 cycles of charge/discharge at 2 mA cm −2 still exhibited relatively uniform morphology without overgrowth of lithium dendrites ( Fig. 3a ). In contrast, uneven growth of mossy lithium was clearly visible after 100 cycles when using the electrolyte without Li 2 S 8 ( Fig. 3b ). 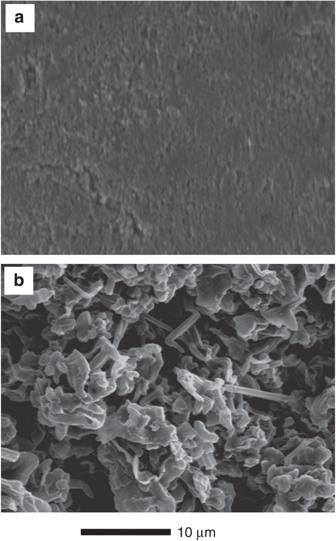Figure 3: Morphology characterization of the surface of the deposited lithium after 100 cycles. SEM images of the top surface of the deposited lithium (edge region) after 100 cycles of charge/discharge at 2 mA cm−2using electrolyte (a) with the addition of both Li2S8(0.18 M) and LiNO3(5 wt%), and (b) with the addition of only LiNO3(5 wt%) at a deposition capacity of 2 mAh cm−2. Figure 3: Morphology characterization of the surface of the deposited lithium after 100 cycles. SEM images of the top surface of the deposited lithium (edge region) after 100 cycles of charge/discharge at 2 mA cm −2 using electrolyte ( a ) with the addition of both Li 2 S 8 (0.18 M) and LiNO 3 (5 wt%), and ( b ) with the addition of only LiNO 3 (5 wt%) at a deposition capacity of 2 mAh cm −2 . Full size image Characterization of the SEI layer As we used bare stainless steel foil as the substrate for lithium deposition, it was also possible to subsequently strip the deposited lithium completely from the substrate, whereupon we observed a thin film attached to the surface of stainless steel foil. This layer is the SEI, which we were able to isolate completely from the lithium metal, unlike previous studies in which the SEI layers are all characterized while on the lithium surface [29] , [30] , [31] , [39] . By isolating the SEI, we were able to accurately investigate the structure and chemical composition of the SEI without interference from metallic lithium. As shown in the SEM images of the SEI layers, the SEI formed in the electrolyte containing only LiNO 3 additive exhibits a porous, cellular morphology ( Fig. 4a ). Moreover, non-uniform SEI layer with lots of cracks and pinholes was also observed using electrolyte with the addition of Li 2 S 8 alone ( Supplementary Fig. 3 ). In contrast, the SEI formed in the electrolyte with both Li 2 S 8 and LiNO 3 showed a mostly planar, uniform layer of SEI with no apparent cracks ( Fig. 4b ). Therefore, we can see that both Li 2 S 8 and LiNO 3 are necessary for the formation of a uniform SEI with high integrity. 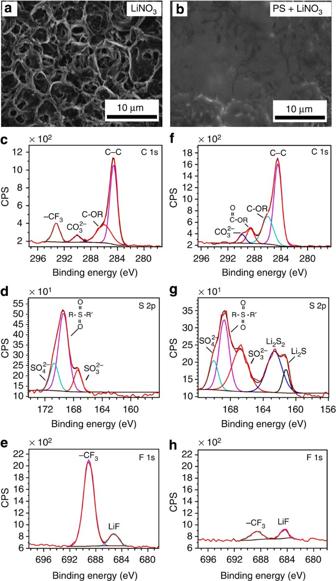Figure 4: Characterization of SEI layers formed in different electrolytes. SEM images of the SEI layers formed in the electrolyte (a) with the addition of only LiNO3(5 wt%) and (b) with the addition of both Li2S8(0.18 M) and LiNO3(5 wt%) after ten cycles (scale bars, 10 μm). X-ray photoelectron spectroscopy (XPS) analysis of the SEI layers, C1s, S2pand F1sspectra are presented, including peak deconvolution and assignments. (c–e) XPS spectra of the SEI layer shown ina.(f–h) XPS spectra of the SEI layer shown inb. PS, lithium polysulfide (Li2S8). Figure 4: Characterization of SEI layers formed in different electrolytes. SEM images of the SEI layers formed in the electrolyte ( a ) with the addition of only LiNO 3 (5 wt%) and ( b ) with the addition of both Li 2 S 8 (0.18 M) and LiNO 3 (5 wt%) after ten cycles (scale bars, 10 μm). X-ray photoelectron spectroscopy (XPS) analysis of the SEI layers, C 1s , S 2p and F 1s spectra are presented, including peak deconvolution and assignments. ( c – e ) XPS spectra of the SEI layer shown in a . (f – h ) XPS spectra of the SEI layer shown in b . PS, lithium polysulfide (Li 2 S 8 ). Full size image We further carried out X-ray photoelectron spectroscopy (XPS) analysis to characterize the chemical compositions of the respective SEIs. Figure 4c–h shows a comparison of the C 1s , S 2p and F 1s spectra of the SEI formed on addition of only LiNO 3 ( Fig. 4c–e ) and on addition of both LiNO 3 and Li 2 S 8 ( Fig. 4f–h ). The spectra presented include the deconvolution of the broad peaks to specific peaks that reflect the various oxidation states of the elements and relevant peak assignments [40] . The binding energies were calibrated with respect to the C 1s peak at 284.5 eV. The differences between the C 1s , S 2p and F 1s spectra of the two samples are clear and pronounced. The major difference lies in the spectra of S 2p . Two extra peaks exist at 161.3 and 162.5 eV for the SEI formed in the electrolyte containing Li 2 S 8 , reflecting the composition of Li 2 S and Li 2 S 2 in the SEI layer. Another distinct difference between the two samples can be found in the C 1s spectra. An extra peak centred at 293.1 eV occurs for the SEI formed in the electrolyte without Li 2 S 8 , whereas this peak does not show up in the SEI formed with electrolyte containing Li 2 S 8 . This peak can be assigned to C in the functional group –CF 3 , which may originate from –CF 3 in Li 2 NSO 2 CF 3 and LiCF 3 . These two compounds are the products of LITFSI decomposition [31] . Moreover, a comparison of the F 1s spectra showed that the signal intensities of the two peaks assigned for F in –CF 3 and LiF (LiF is also a product resulting from LITFSI decomposition [31] ) for the SEI formed in the electrolyte containing Li 2 S 8 are weaker than those formed in the electrolyte without Li 2 S 8 . It is noted that in the F 1s spectra, the intensity of the peak for –CF 3 is greatly suppressed with addition of both LiNO 3 and Li 2 S 8 , whereas the intensity of the peak for LiF is slightly weaker than the one when only LiNO 3 is present. This indicates that the presence of both LiNO 3 and Li 2 S 8 greatly reduced the degradation reactions that lead to the formation of LiCF 3 and Li 2 NSO 2 CF 3 rather than suppressed the one that leads to LiF. Recent research from Archer and colleagues [28] showed that adding LiF suspensions into the electrolyte could effectively suppress the lithium dendrites growth. In our experiment, the LiF detected from the SEI layer was formed due to the LITFSI decomposition and the amount of LiF generated was very limited. Therefore, it could not play a significant role in preventing the dendrites growth as shown in the paper by Archer and colleagues [28] . As to the N 1s spectra ( Supplementary Fig. 4 ), for both samples, the three peaks centred at 399.9, 404.3 and 408.0 eV can be assigned to N in the N–S bond, NO 2 − and NO 3 − , respectively, indicating that LiNO 3 is reduced by lithium to LiNO 2 , whereas the sulfone species in the LITFSI can be oxidized to SO 3 2− and SO 4 2− (identified from the S 2p spectra for both samples). The difference in the N 1s spectra of the two samples is that the N 1s signal for the SEI containing Li 2 S/Li 2 S 2 is much weaker, only slightly higher than noise level. Cycling stability and Coulombic efficiency The Coulombic efficiency was examined using our two-electrode coin cell design, calculated as the amount of lithium stripped (calculated based on the capacity extracted) divided by the amount of lithium plated (calculated based on the capacity deposited) on the stainless steel foil. Unlike symmetric cells that use two electrodes of lithium foil that are essentially infinite sources for lithium [29] , [30] , [31] , [39] , our design allows the lithium loss on cycling to be accurately determined. As the cycle life of lithium metal electrodes can be correlated with electrolyte decomposition [11] , [12] , [30] , the same amount of electrolyte (30 μl) was used in each cell. 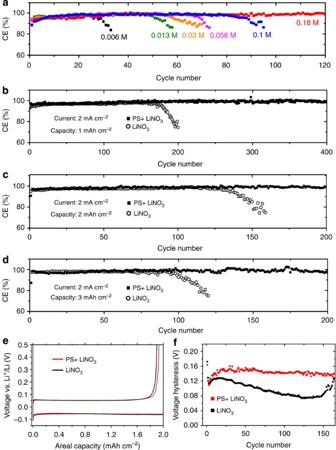Figure 5: Electrochemical characterization of the electrodes for lithium deposition/dissolution. (a) Coulombic efficiency of the cells versus cycle number using electrolytes containing different concentrations of Li2S8at a current density of 2.0 mA cm−2with a constant lithium deposition capacity of 2.0 mAh cm−2(the LiNO3additives in these electrolytes are all 1 wt%,∼0.15 M). (b–d) Cycling performances of the cells using electrolyte containing 0.18 M Li2S8and 5 wt% LiNO3(∼0.75 M, close to the saturation concentration of LiNO3in 1,3-dioxolane/1,2-dimethoxyethane (DOL/DME) electrolyte) at a current density of 2.0 mA cm−2with a deposition capacity of 1, 2 and 3 mAh cm−2, respectively. The hollow symbols represent data of the control samples using electrolyte with 5 wt% LiNO3. Comparison of (e) voltage profiles and (f) average voltage hysteresis of the lithium deposition/dissolution process with lithium metal as the reference/counter electrode at 2 mA cm−2using electrolyte containing only LiNO3(5 wt%) (black line/square) and containing both Li2S8(0.18 M) and LiNO3(5 wt%) (red line/square). The voltage profiles are obtained at the second cycle of lithium deposition/dissolution. PS, lithium polysulfide (Li2S8). Figure 5a shows the Coulombic efficiency versus cycle number of cells containing electrolyte with different concentrations of Li 2 S 8 , all tested at a current density of 2.0 mA cm −2 and a constant lithium deposition capacity of 2.0 mAh cm −2 . The LiNO 3 concentration used throughout was 1 wt% ( ∼ 0.15 M). It can be seen that the cycle life increases with increasing concentration of polysulfide. When the concentration of Li 2 S 8 in the electrolyte is increased to 0.18 M, the Coulombic efficiency is ∼ 99.4% after 120 cycles (average Coulombic efficiency over 120 cycles is ∼ 98.1%), whereas for 1 wt% LiNO 3 alone the efficiency decreases to <90% after just 45 cycles (average Coulombic efficiency over the first 40 cycles is ∼ 95.6%, Supplementary Fig. 5 ). These results clearly demonstrate that the polysulfide concentration in the electrolyte is critical to the formation of a highly stable SEI. We believe that enough polysulfide must be present to form a uniform protective surface film containing Li 2 S/Li 2 S 2 (as demonstrated in Fig. 4 ) during the first few cycles, which then blocks further contact and continuous reaction between lithium and the electrolyte. In comparison, the SEI formed in the electrolyte containing a low concentration of Li 2 S 8 (0.013 M) exhibited a similar morphology to that in Fig. 4a , in which the distribution of Li 2 S/Li 2 S 2 is not uniform enough to cover the entire surface of the SEI and prevent further electrolyte decomposition and dendrite growth (SEM image, Supplementary Fig. 6 ). In addition, the Coulombic efficiency versus cycle number of cell containing electrolyte with the addition of Li 2 S 8 (0.18 M) alone was also investigated ( Supplementary Fig. 7 ): the Coulombic efficiency was very low, only ∼ 80%, and decreased to 40% after 50 cycles, indicating the vigorous reaction between lithium and Li 2 S 8 . This also, on the other hand, explains why Li 2 S 8 alone could not enable the formation of a homogeneous SEI and reduce the electrolyte decomposition. We also found that the cycle life and Coulombic efficiency can be slightly improved by increasing the concentration of LiNO 3 . When the amount of LiNO 3 was increased from 1 to 2.5 wt%, the cell can last for about 60 cycles with average Coulombic efficiency of ∼ 96.5% ( Supplementary Fig. 5 ). Figure 5: Electrochemical characterization of the electrodes for lithium deposition/dissolution. ( a ) Coulombic efficiency of the cells versus cycle number using electrolytes containing different concentrations of Li 2 S 8 at a current density of 2.0 mA cm −2 with a constant lithium deposition capacity of 2.0 mAh cm −2 (the LiNO 3 additives in these electrolytes are all 1 wt%, ∼ 0.15 M). ( b – d ) Cycling performances of the cells using electrolyte containing 0.18 M Li 2 S 8 and 5 wt% LiNO 3 ( ∼ 0.75 M, close to the saturation concentration of LiNO 3 in 1,3-dioxolane/1,2-dimethoxyethane (DOL/DME) electrolyte) at a current density of 2.0 mA cm −2 with a deposition capacity of 1, 2 and 3 mAh cm −2 , respectively. The hollow symbols represent data of the control samples using electrolyte with 5 wt% LiNO 3 . Comparison of ( e ) voltage profiles and ( f ) average voltage hysteresis of the lithium deposition/dissolution process with lithium metal as the reference/counter electrode at 2 mA cm −2 using electrolyte containing only LiNO 3 (5 wt%) (black line/square) and containing both Li 2 S 8 (0.18 M) and LiNO 3 (5 wt%) (red line/square). The voltage profiles are obtained at the second cycle of lithium deposition/dissolution. PS, lithium polysulfide (Li 2 S 8 ). Full size image Figure 5b–d compares the cycling performance of cells tested at the same current density of 2.0 mA cm −2 , but cycled to different deposition capacities of 1, 2 and 3 mAh cm −2 , respectively. The solid symbols represent data of the cells using electrolyte containing both 0.18 M Li 2 S 8 and 5 wt% LiNO 3 ( ∼ 0.75 M, close to the saturation concentration of LiNO 3 in 1,3-dioxolane /1,2-dimethoxyethane electrolyte), whereas the hollow symbols represent data of the control samples using electrolyte with 5 wt% LiNO 3 alone. At deposition capacity of 1 mAh cm −2 ( Fig. 5b ) over the cycling range from 100 to 400 cycles, the cell maintains a high average Coulombic efficiency of 99.1%. In contrast, when using electrolyte containing only the 5 wt% LiNO 3 , the Coulombic efficiency drops to <92% after 180 cycles. Even when the capacity is increased to 2 and 3 mAh cm −2 ( Fig. 5c,d ), the Coulombic efficiency with polysulfide additive has an average value of ∼ 98.5% over 200 cycles (and is higher at ∼ 99.0% between 70 and 200 cycles), whereas the Coulombic efficiencies without polysulfide decreased to <92% after 140 and 102 cycles at deposition capacity of 2 and 3 mAh cm −2 , respectively. The formation of a stable SEI is also reflected in cell polarization and its evolution with cycling. Figure 5e shows voltage profiles during the second cycle of cells with and without polysulfide additive, measured at 2 mA cm −2 . It can be observed that the polarization of the two cells at this stage of cycling is nearly identical. Figure 5f shows the average voltage hysteresis versus cycle number. For the cell using electrolyte-containing polysulfide, the voltage hysteresis in the lithium deposition/dissolution first slightly increases as the SEI layer is formed, but then remains almost unchanged at ∼ 145 mV over the remaining cycles, demonstrating its high stability. In comparison, the cell without polysulfide shows behaviour that is characteristic of dendrite formation. The voltage hysteresis first decreases as the cycle number increases, which can be attributed to the creation of greater lithium surface area and therefore lower total resistance. However, with continued cycling the voltage hysteresis suddenly increases, which is due to the loss of electrolyte caused by electrolyte decomposition. In addition, we further tested the influence of Li 2 S 8 on electrolyte conductivity and interfacial resistance via electrochemical impedance spectroscopy measurements using lithium-metal symmetrical coin cells ( Supplementary Fig. 8 and Supplementary Note 1 ). We found that the ionic conductivity did not change a lot by adding the polysulfide (0.18 M) into the electrolyte. The ionic conductivity decreased a little bit from 3.49 to 3.21 mS cm −1 after adding the polysulfide (see calculation in Supplementary Information). The interfacial resistance, on the other hand, increased from 9 to 67 Ω due to the formation of the SEI that comprises Li 2 S 2 /Li 2 S. However, this increase of the interfacial impedance did not have significant influence on the lithium deposition/stripping process at a current of 2 mA cm −2 as shown in Fig. 5e . In-situ optical microscopy study of lithium metal deposition We further used in-situ optical microscopy to characterize the process of lithium deposition. We designed a quartz cell housing with transparent windows and a rectangle cavity inside ( Fig. 6a ), in which a sandwich structure of lithium metal, separator and stainless steel substrate was assembled. The fabricated cell was mounted on the optical microscope stage with the transparent window facing the lens for in-situ characterization. Lithium dendrite growth on the stainless steel surface was recorded during lithium deposition at a current density of 5 mA cm −2 . 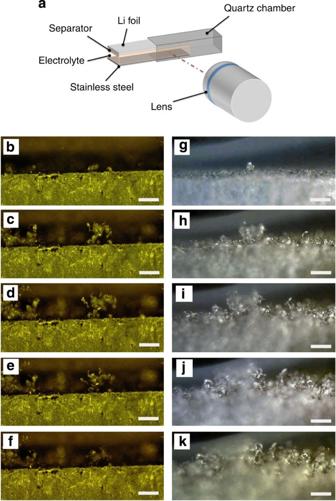Figure 6:In-situoptical microscopy study of lithium dendrite formation. (a) Schematic illustration of the quartz cell device with transparent windows and rectangle empty space inside as the cell housing, in which a sandwich structure of lithium metal, separator and stainless steel substrate was assembled. The fabricated cell was put on the stage of optical spectroscopy with transparent window facing to the lens forin-situcharacterization. (b–f) A series of dark-field optical microscope images of the cell’s cross-section (b–f, optical images versus increasing lithium deposition time), revealing the growing process of lithium dendrites at 5 mA cm−2on the stainless steel substrate using electrolyte with the addition of both Li2S8and LiNO3. (g–k) A series of dark-field optical microscope images of the cell’s cross-section (g–k, optical images versus increasing lithium deposition time), showing the growing process of lithium dendrites using electrolyte with the addition of only LiNO3at the same current density asb–f. Scale bar, 100 μm. Figure 6b–f,g–k shows a series of dark-field optical microscope images of the cell’s cross-section (each column: optical images versus increasing lithium deposition time), revealing the difference in the growing process of lithium dendrites on the stainless steel substrate using electrolyte with and without the addition of polysulfide, respectively (videos of the growth process, see Supplementary Movie 1 and 2 ). As shown in Fig. 6b–f , we observed that the lithium dendrites formed in the polysulfide-containing electrolyte first grew then shrank, clearly revealing chemical etching of the dendrites by reaction with the lithium polysulfide. In comparison, when using electrolyte without polysulfide ( Fig. 6g–k ), the lithium dendrites grew continuously throughout the experiment. Figure 6: In-situ optical microscopy study of lithium dendrite formation. ( a ) Schematic illustration of the quartz cell device with transparent windows and rectangle empty space inside as the cell housing, in which a sandwich structure of lithium metal, separator and stainless steel substrate was assembled. The fabricated cell was put on the stage of optical spectroscopy with transparent window facing to the lens for in-situ characterization. ( b – f ) A series of dark-field optical microscope images of the cell’s cross-section ( b – f , optical images versus increasing lithium deposition time), revealing the growing process of lithium dendrites at 5 mA cm −2 on the stainless steel substrate using electrolyte with the addition of both Li 2 S 8 and LiNO 3 . ( g – k ) A series of dark-field optical microscope images of the cell’s cross-section ( g – k , optical images versus increasing lithium deposition time), showing the growing process of lithium dendrites using electrolyte with the addition of only LiNO 3 at the same current density as b – f . Scale bar, 100 μm. Full size image To reveal the mechanism why a combined effect of LiNO 3 and Li 2 S 8 can contribute to the formation of a uniform SEI layer, we further conducted XPS analysis on the composition of the SEI formed in the electrolyte with the addition of Li 2 S 8 alone ( Supplementary Fig. 3 ). It was found that this SEI layer could not prevent electrolyte decomposition: strong –CF 3 peak was detected from the C 1s and F 1s spectra, which is similar to the case with the addition of LiNO 3 alone ( Fig. 4c–e ). This finding is consistent with a previous study reported by Zu and Manthiram [41] , showing that the passivation by bulk-insulating Li 2 S particles reduced from Li 2 S x caused heterogeneities of the lithium metal surface and thus aggravated lithium dendrite formation. When we added both LiNO 3 and Li 2 S 8 into the electrolyte, in combination with what we observed from the SEM and XPS results, we assume that there could be a competing effect between these two additives towards the reaction with lithium metal, in which LiNO 3 could first react with lithium metal and help to passivate the lithium metal surface to reduce the extent of the reaction between Li 2 S 8 and lithium. In this case, Li 2 S/Li 2 S 2 could mainly form in the upper layer of the SEI, acting as a protective layer to minimize the electrolyte from decomposition, contributing to longer cycle life and superior Coulombic efficiency. Based on the mechanism we discussed above, other polysulfide such as Li 2 S 6 and Li 2 S 4 , which can also be reduced to Li 2 S 2 /Li 2 S, could also have similar effect to reinforce the formation of a uniform and stable SEI layer when combined with LiNO 3 . In conclusion, we have demonstrated that lithium dendrite growth can be effectively suppressed via manipulating the chemical reactions of lithium, lithium polysulfide and LiNO 3 . By controlling the concentration of polysulfide and LiNO 3 in the electrolyte, a stable and uniform SEI can be formed on the lithium surface, which greatly minimizes electrolyte decomposition and prevents dendrite growth. Observations were made at the edge regions of the deposition area, where dendrite growth is most exaggerated due to the absence of physical constraint. In practical lithium-ion cells, this is also the region most susceptible to lithium dendrite formation on fast charging and during long-term cycling. We found that no lithium dendrites formed at a practical current density of 2 mA cm −2 up to a deposited lithium capacity of 6 mAh cm −2 , which is about twice the area capacity of current commercial lithium-ion battery electrodes. The Coulombic efficiency and cycle life of the lithium metal cells using electrolyte-containing polysulfide are significantly improved, with Coulombic efficiency being maintained at ∼ 99% for over 300 cycles at 2 mA cm −2 . In addition, direct observations of dendrite formation using in-situ optical imaging showed the dissolution of initially formed dendrites even as overall deposition proceeded. Our findings show that the reaction that has long been considered a critical flaw in lithium–sulfur batteries can actually benefit lithium metal-based battery systems when it is properly controlled. This illustrates a new strategy for solving dendrite issues associated with lithium metal anodes, which could be applied to next-generation high-energy-density battery systems such as lithium–sulfur and lithium–air batteries, as well as other metal–anode battery chemistries. Electrochemical measurements Galvanostatic experiments were performed using a 96-channel battery tester (Arbin Instrument). The electrolyte is 1 M LiTFSI in 1,3-dioxolane and 1,2-dimethoxyethane (volume ratio 1:1). Different amounts of lithium nitrate and lithium polysulfide (Li 2 S 8 ) were added to the electrolyte as additives and thus systematically tested. The Li 2 S 8 solution was prepared through a chemical reaction between sulfur and lithium sulfide based on our previous report [42] . The process of lithium metal plating/stripping was investigated using a two-electrode configuration assembled in the 2,032-type coin cells (MTI Corporation), which is composed of a lithium metal electrode and a stainless steel foil (substrate for lithium plating/stripping). A constant current is applied to the electrodes, while the potential is recorded versus time. A fixed amount of lithium is first deposited onto the stainless steel substrate followed by subsequent process of lithium dissolution and re-deposition. Coulombic efficiency is calculated by dividing the amount of lithium stripped by the amount of lithium plated on the stainless steel foil during each cycle. The electrolyte conductivity and interfacial resistance is tested via electrochemical impedance spectroscopy measurements using lithium metal symmetrical coin cells. Characterization SEM images were taken using FEI XL30 Sirion SEM operated at an accelerating voltage of 5 kV. The electronic environment of the SEI layers was investigated through XPS (Phi5000 VersaProbe, Ulvac-Phi) with Al Kα radiation. In-situ optical microscopy study was carried out using a quartz cell with transparent windows and rectangle empty space inside as the cell housing, in which a sandwich structure of lithium metal, separator and stainless steel substrate was assembled. The fabricated cell was put on the stage of optical spectroscopy with transparent window facing to the lens for in-situ characterization. The lithium dendrite growth on the stainless steel surface was recorded in real time during lithium deposition. How to cite this article: Li, W. et al. The synergetic effect of lithium polysulfide and lithium nitrate to prevent lithium dendrite growth. Nat. Commun. 6:7436 doi: 10.1038/ncomms8436 (2015).